In situatomic-scale observation of continuous and reversible lattice deformation beyond the elastic limit The elastic strain sustainable in crystal lattices is usually limited by the onset of inelastic yielding mediated by discrete dislocation activity, displacive deformation twinning and stress-induced phase transformations, or fracture associated with flaws. Here we report a continuous and gradual lattice deformation in bending nickel nanowires to a reversible shear strain as high as 34.6%, which is approximately four times that of the theoretical elastic strain limit for unconstrained loading. The functioning deformation mechanism was revealed on the atomic scale by an in situ nanowire bending experiments inside a transmission electron microscope. The complete continuous lattice straining process of crystals has been witnessed in its entirety for the straining path, which starts from the face-centred cubic lattice, transitions through the orthogonal path to reach a body-centred tetragonal structure and finally to a re-oriented face-centred cubic structure. The theoretical elastic limit at which a perfect crystal becomes mechanically unstable is the upper bound of the achievable strength and elastic strain of a material. Under uniaxial loading of bulk samples, the maximum elastic strain that can be achieved in the lattice is normally no larger than ~0.2%, which is limited by the onset of inelastic yielding mediated by discrete dislocation activities [1] , deformation twinning [2] and stress-induced phase transformations [3] , or by intervention due to fracture associated with flaws [1] . By reducing material dimensions to the micrometre or even nanometre regime, large reversible lattice strains of ~2 to 8%, close to the theoretical limit, have been observed in ‘defect-free’ whiskers [4] , [5] , [6] , micro-pillars [7] , [8] , [9] , [10] , [11] and nanowires (NWs) [12] , [13] . However, if inelastic events associated with dislocations [14] , [15] , cracking [16] , twinning [2] and first-order phase transitions [17] , [18] can be largely suppressed under confining loading conditions in small regions, a continuous and reversible lattice strain beyond ~8% may become possible. The upper limit of lattice strain is of obvious interest in materials science and physics. Theorists have attempted to compute it from atomistic models since the 1920s [19] , [20] , [21] , [22] . Such estimates predicted that the upper limit of lattice deformation strain in metals can surpass 30% [23] , [24] , but it has never been observed in experiments. In this paper, we report in situ bending experiments of nickel (Ni) NWs inside a transmission electron microscope (TEM), and provide direct and atomic-scale experimental evidence that the theoretically predicted continuous lattice shear strain, which is as large as 34.6%, can be indeed sustained in a confined crystalline lattice. The continuous lattice shearing can be, however, terminated at strains lower than 34.6%, due to defect generation. With the release of the stored ultra-large elastic energy, the highly strained lattices may be forced to recover to their original shape. This in situ bending experiment of Ni NWs allowed us to observe, for the first time, the entire and the reversible continuous path of the face-centred cubic (FCC) lattice, transitions through the orthogonal path to reach a body-centred tetragonal (BCT) structure and finally to a re-oriented face-centred (FCC R ) cubic structure. In situ bending deformation of NWs Ni NWs were synthesized using an electrochemical deposition method [25] . TEM micrographs showed that the as-prepared Ni NWs had an FCC structure and consisted of parallel (111) twin lamellae. The nanotwin-structured Ni NWs are ~50 μm in length and 30–50 nm in diameter ( d ). The growth direction of the NWs was nearly parallel to the [112] crystal orientation ( Supplementary Fig. S1 ). The NWs were randomly spread to bridge on a pre-broken colloidal thin film (CTF) on a TEM specimen grid (see Fig. 1a–c ). The scattered NWs could then be bent or stretched controllably by expansion or contraction of the CTFs under the irradiation of an electron beam (see Supplementary Movie 1 and Supplementary Methods section or the studies by Zheng et al. [26] and Wang et al. [27] for details). The entire NW bending experiments were conducted inside a TEM, but in the absence of direct electron-beam irradiation on the NWs during straining. 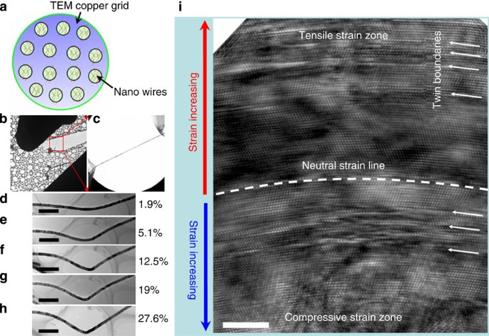Figure 1:In situbending of individual twin-structured Ni NWs. (a) A schematic view shows that the Ni NWs were scattered on the previously broken TEM grid, which was covered by CTFs. (b) An example shows that a single NW could be deformed by tensile stress induced by the CTFs under electron-beam irradiation. (c) Enlarged TEM image taken from the red framed region of (b). (d–h) A series of TEM images that shows the bending process of a single Ni NW. The strain sustained by the Ni NW increased from 1.9% to 27.6%. (i) Atomic-scale image of the bent Ni nanowire. The dotted white line indicates the neutral axis, showing the highly bent arc-shaped (111) lattices. The bent TB is marked with white arrows. The dimensions of the scale bars are: (d–h), 100 nm; (i), 2 nm. Figure 1d–h shows a series of TEM images depicting the continuous bending process of a Ni NW ( d ~35 nm); the effective average strain rate was ~10 −4 s −1 . By monitoring the bending angle of the Ni NW as a function of the time elapsed in the bending experiment ( Fig. 1d–h ), we observed and monitored the continuous bending deformation of the NW; the global strain experienced by the NW changed from the initial 1.9% ( Fig. 1d ) to a final ~27.6%. Figure 1: In situ bending of individual twin-structured Ni NWs. ( a ) A schematic view shows that the Ni NWs were scattered on the previously broken TEM grid, which was covered by CTFs. ( b ) An example shows that a single NW could be deformed by tensile stress induced by the CTFs under electron-beam irradiation. ( c ) Enlarged TEM image taken from the red framed region of ( b ). ( d – h ) A series of TEM images that shows the bending process of a single Ni NW. The strain sustained by the Ni NW increased from 1.9% to 27.6%. ( i ) Atomic-scale image of the bent Ni nanowire. The dotted white line indicates the neutral axis, showing the highly bent arc-shaped (111) lattices. The bent TB is marked with white arrows. The dimensions of the scale bars are: ( d – h ), 100 nm; ( i ), 2 nm. Full size image Using the newly developed atomic-scale imaging and straining technique [26] , [27] , the atomic-scale deformation mechanisms of the NWs could be directly observed. Figure 1 i shows a snapshot of the time- and position-resolved atomic-scale image of the bent Ni NW. The highly bent arc-shaped (111) lattices and twin boundaries (TB) are highlighted by a dotted white line. These twin platelets are thin slabs with thicknesses of 1–6 nm. The dotted white line indicates the neutral axis, whose longitudinal strain is close to zero. The regions above this neutral line sustain tensile strains, whereas the areas below this neutral axis line are subjected to compressive strains. The dynamic atomic-scale characterization is thus able to record the lattice strain evolution of the bent Ni NW and related elastic–plastic transformation process at the atomic scale in situ and in real time. Ultra-large continuous lattice strain The ultra-large lattice strain can be frequently observed in the bent Ni NWs. 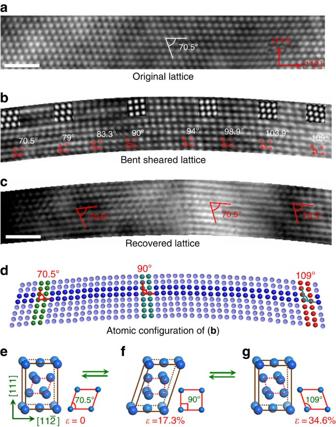Figure 2: Continuous and reversible lattice strain beyond the elastic limit. (a) HRTEM image of a Ni nanowire captured when the bent strain is ~1.9%. (b) Enlarged atomic-scale image shows the continuous increase inαfrom 71° to ~109°. The simulated HREM images are inserted accordingly. (c) HRTEM image captured after the strain released. No square lattice and other type sheared lattices were observed, indicated the 34.6% lattice shear strain was fully recovered. (d) Atomic configurations corresponding to (b) to show the ultra-large continues lattice shear from 0 to 34.6%. (e–g) Schematic 3D structures and corresponding side views show the shear and recover process of the FCC lattice. The scale bars are for 1 nm. Figure 2 shows, on the atomic scale, how bending induces a continuous lattice strain along the axial direction. The high-resolution TEM (HRTEM) micrographs show that the inter-planar angle ( α ) of the {111} planes continuously changes from the normal 70.5° (projected along the [110] direction of the FCC lattice) to ~90° and to 109° (also see other example of Supplementary Fig. S2 ). This in situ atomic observation demonstrates that the inter-planar angle α of the {111} planes in the bent NW continuously increased to exceed 90° and approached that corresponding to theoretical lattice shearing limit, that is, ~109°. Figure 2a is a typical atomic-scale image of the initial atomic structure of the Ni NW. Figure 2b is an atomic image showing that the dislocation-free (see Supplementary Fig. S3 ) lattice shear gives rise to the gradual increase in α from ~70.5° to ~90° and then to ~109°, which corresponds to the continuous lattice shear strain from 0% to 17.3% and further to 34.6%. This large shear strain accomplishes the continuous lattice changes from the original FCC, through the orthogonal path, to the tetragonal lattice and finally, to a FCC R ( Supplementary Fig. S4 ).This matches well with our ab initio simulation (see in Fig. 4 below) and the related HRTEM image simulation (see Supplementary Figs S5 and S6 ). Interestingly, the ultra-large lattice shear is fully reversible. When further straining was imposed, the continuous lattice shearing was terminated by dislocations/small angle boundaries. The large elastic energy stored in the lattices was thus released and it effectively forced all of the sheared lattices including the FCC R lattice (with strain of 34.6%) back to the original FCC lattice. This is shown in Fig. 2c where the lattices return to their original parallelogram shape, with α ~70.5° corresponding to the original FCC lattice. Figure 2d is a schematic drawing of the projected atomic configurations corresponding to the HRTEM images of Fig. 2b to show the FCC structure with the shear strains of 0, 17.3 and 34.6% more clearly. The two arrays of dark-blue dots present the continuous lattice strain in the bent Ni NW. The green atomic columns show the original FCC lattice while the teal columns correspond to the lattice shearing with ~17.3% strain and the red ones display the 109° sheared atomic columns. Derived from Fig. 2a–d , Fig. 2e–g illustrates the three-dimensional (3D) structures and side views of the FCC lattice with shear strains of 0, 17.3 and 34.6%, respectively. The arrows indicate the lattice shearing process and the recovering route. This ultra-large continuous lattice shear was only observed in 1–4 nm thickness twin lamellae that sustain the complex strain in the bent NWs. The region that has undergone the lattice change was as large as 4 nm × 10 nm in size. The lattices in the compressive region were distorted and no obvious shear was observed ( Supplementary Fig. S7 ). Figure 2: Continuous and reversible lattice strain beyond the elastic limit. ( a ) HRTEM image of a Ni nanowire captured when the bent strain is ~1.9%. ( b ) Enlarged atomic-scale image shows the continuous increase in α from 71° to ~109°. The simulated HREM images are inserted accordingly. ( c ) HRTEM image captured after the strain released. No square lattice and other type sheared lattices were observed, indicated the 34.6% lattice shear strain was fully recovered. ( d ) Atomic configurations corresponding to ( b ) to show the ultra-large continues lattice shear from 0 to 34.6%. ( e – g ) Schematic 3D structures and corresponding side views show the shear and recover process of the FCC lattice. The scale bars are for 1 nm. 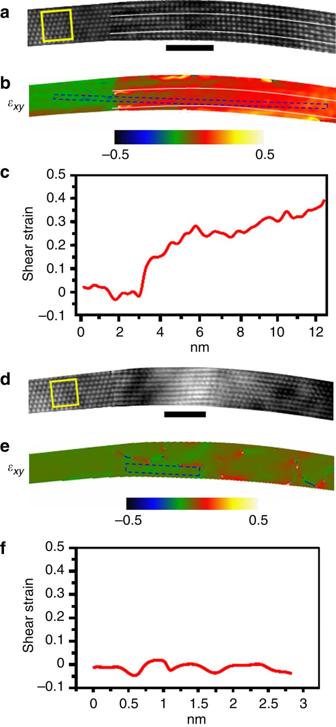Figure 3: Shear strain distribution from GPA. (a) The composite HRTEM image created by mergingFig. 2a,b, the left side corresponding toFig. 2aand the right side corresponding toFig. 2b. The unstrained lattice such as yellow framed region serves as a reference. (b) The corresponding shear strain map (ɛxy) of (a) and the colour variation from black to yellow indicates the variation of shear strain values from −0.5 to 0.5. (c) Quantitative shear strains extracted from the blue dashed-line framed region of (b) by using intensity line scanning from left to right (line width 0.4 nm). (d) The composite HRTEM image created by mergingFig. 2a,c. (e) The corresponding shear strain map (ɛxy) of (f). (f) Typical quantitative shear strains extracted from the blue dashed-line framed region of (e) by using intensity line scanning from left to right (line width 0.6 nm). The scale bars are for 2 nm. Full size image Figure 3: Shear strain distribution from GPA. ( a ) The composite HRTEM image created by merging Fig. 2a,b , the left side corresponding to Fig. 2a and the right side corresponding to Fig. 2b . The unstrained lattice such as yellow framed region serves as a reference. ( b ) The corresponding shear strain map ( ɛ xy ) of ( a ) and the colour variation from black to yellow indicates the variation of shear strain values from −0.5 to 0.5. ( c ) Quantitative shear strains extracted from the blue dashed-line framed region of ( b ) by using intensity line scanning from left to right (line width 0.4 nm). ( d ) The composite HRTEM image created by merging Fig. 2a,c . ( e ) The corresponding shear strain map ( ɛ xy ) of ( f ). ( f ) Typical quantitative shear strains extracted from the blue dashed-line framed region of ( e ) by using intensity line scanning from left to right (line width 0.6 nm). The scale bars are for 2 nm. 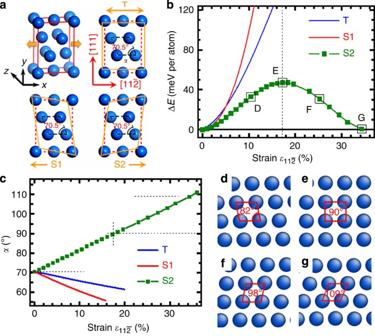Figure 4:Ab initiosimulation of the continuous lattice deformation. (a) A 3D structure of asupercell and the side views of the FCC that is tensile along thedirection (T), shear along(S1) and(S2) directions. (b,c) Calculated energy changes and inter-plane lattice angleα(as denoted inFig. 3a) as a function of the strain. The red line indicates the energy as a function of the tensile strain, the green line indicates the energy as a function of the shear strain alongand blue squares indicate the energy as a function of the shear strain along. The energy saddle point (maximum energy marked ‘E‘) corresponds to the BCT structure in our TEM observation.(d–g) The atomic configuration projections in theplane and the corresponding strains are 0.115, 0.173, 0.25 and 0.346, respectively. Full size image Figure 4: Ab initio simulation of the continuous lattice deformation. ( a ) A 3D structure of a supercell and the side views of the FCC that is tensile along the direction (T), shear along (S1) and (S2) directions. ( b , c ) Calculated energy changes and inter-plane lattice angle α (as denoted in Fig. 3a ) as a function of the strain. The red line indicates the energy as a function of the tensile strain, the green line indicates the energy as a function of the shear strain along and blue squares indicate the energy as a function of the shear strain along . The energy saddle point (maximum energy marked ‘ E ‘) corresponds to the BCT structure in our TEM observation. ( d – g ) The atomic configuration projections in the plane and the corresponding strains are 0.115, 0.173, 0.25 and 0.346, respectively. Full size image Atomic-scale spatial distribution of the continuous lattice strain The accurate strain distribution in the NWs can be directly mapped at the atomic scale from HRTEM images by using the geometrical phase analysis (GPA) [28] , [29] or peak-pair analysis method [30] , [31] . Here the GPA technique is used to quantify the local lattice shear strain of the bent Ni NW as shown in Fig. 3 . The GPA generates quantitative strain maps from standard HRTEM images [28] , [30] and has been used previously in quantifying the strains in NWs [28] , [29] , [30] , [31] . Here we merge Fig. 2a–c to create new composite HRTEM images for GPA analysis. This method can provide a larger unstrained area as the reference for precise strain mapping. As shown in Fig. 3a , the right side of the HRTEM image is corresponding to Fig. 2b , in which the lattice-angle α continuously shears from 70.5° to 109°. The yellow framed region in the left side of Fig. 3a was defined as a reference region with zero strain. This region has been confirmed to be free of dislocations ( Supplementary Fig. S3 ). Figure 3b shows the GPA shear strain (along the direction) maps of ɛ xy (for the strain maps of ɛ xx and ɛ yy see Supplementary Fig. S8 ), the colour variation from dark blue to bright yellow corresponds to the strains from −0.5 to 0.5. The quantitative shear strains, extracted from the coloured strain maps using intensity line scanning, are shown in Fig. 3c . From left to right, the shear strains increase from 0 ( α =70.5°) to ~35% ( α =109°), consistent with the shear angle analysis and the ab initio simulations, which will be shown below in detail. Furthermore, the unstrained regions have negligible strain values, indicating that the procedure adopted is accurate (see Supplementary Figs S8 and S9 ). We also map the shear strains using the local lattice as the reference and they show the same trend ( Supplementary Fig. S10 ). The GPA analysis was also performed for the HRTEM image with the strain released. Figure 3d is the composite HRTEM image that was created by merging Fig. 2a,c . The corresponding shear strain maps are shown in Fig. 3e . The sharp contrast observed in the strain maps was caused by intervention of dislocations. Most of the regions show low strain values with green colours. This is confirmed by the typical quantitative shear strain plot shown in Fig. 3f . The strain was extracted from the blue dashed-line framed region of Fig. 3e using the intensity line scanning from left to right (line width 0.6 nm). We have also examined other regions using intensity line scans, and the results show that the strain is very low in the lattice-recovered NW, except in those regions near the dislocation core ( Supplementary Figs S8 and S9 ). Ab initio simulation We simulated the lattice structure evolution by straining an FCC unit cell along the direction. The stress direction is the same as that in our in situ TEM experiments. As shown in Fig. 4a , three typical deformation routes were selected, including the uniaxial tensile along direction (T), shearing along direction (S1) and direction (S2). The calculated strain–energy curves are shown in Fig. 4b . It indicates that the shear is the most energetically favourable deformation route, that is, the lowest energy path. The inter-plane lattice angle α as a function of strain is shown in Fig. 4c . In fact, only the route of shearing along direction is consistent with our HRTEM observation, in which, the inter-plane lattice angle monotonically changes from 70.5° to ~109° on increasing the shear strain. Although the ideal shear strain in the FCC lattice has been predicted for many years [19] , [20] , [21] , [22] , [23] , [24] , the current study is the first experimental demonstration that the theoretically predicted ideal lattice shear can be realised, indeed, in actuality when dislocation and twin activities are completely suppressed. Although the atomic structure is revealed by the phase-contrast HRTEM in this study, the continuous lattice shear in the system <112>{111} is fully supported by the excellent match between the HRTEM observation, HRTEM image simulation and ab initio simulation of the lattice structure and corresponding straining process ( Fig. 4c–g) . The simulation provides more details regarding the physical understanding of the achieved maximum strain of 34.6%. As shown in Fig. 4b , the total energy of the strained unit cell along the shear path monotonically increases with strain until it reaches the maximum at ~17.3% strain, and then monotonically decreases with the further increase of strain to the minimum at the strain of ~34.6%. Through the orthogonal lattice straining path (highly strained FCC structure, see Supplementary Fig. S4 ), the unit cell at the first saddle point can be described by a BCT structure ( a t = c t =2.86 Å, b t =2.62 Å) with the maximum and the {111} inter-plane lattice angle α =90°. Relative to the original FCC lattice, the resultant strain is 17.3% at the saddle point. The unit cell at the second saddle points has the FCC structure with a =3.49 Å but an inter-plane lattice angle α =109° (a FCC R structure), whereas the resultant strain is 34.6%, corresponding to the original FCC. The main lattice parameters were obtained by ab initio simulation ( Supplementary Table S1 ). For coarse-grained materials, yielding occurs at a very low strain of 0.2%; in nano-grained metals, elastic deformation by continuous lattice straining may extend to ~1% [32] . But in all cases, the lattice strains in these materials are small, limited by the activation of dislocations and deformation twins at a low stress level (for example, hundreds of MPa). For whiskers and NWs, the lattice can reach an elastic strain as high as ~8% [4] , [7] , [12] , [13] , but in uniaxial loading conditions, the continuous lattice strain (elastic strain) has never reached >8%. Our observation of 34.6% is in fact four times as large as the ideal elastic limit in normal conditions. This is because all the inelastic events have been completely suppressed by confinement and size effect. More specifically, the extraordinary straining capability in bending Ni NWs arises for several reasons. First, besides the fact that perfect TB can serve as a strong dislocation obstacle to keep away the dislocations nucleated from the free surface [33] , [34] , the 1–6-nm-thick twin slabs in the twin-structured NWs approach the predicted size limit where the normal full and partial dislocation activities can be almost entirely suppressed. As shown in Supplementary Fig. S1 , the original growth TB separates the NWs into a small isolated region (1–6 nm), and the large lattice shear-strained region only appeared in the 1–4 nm thickness twin. The critical shear stresses needed to nucleate a perfect dislocation and partial dislocation can be calculated according the formula [1] , [35] : and here, τ N and τ P are the critical shear stresses needed to nucleate a perfect dislocation and partial dislocation, respectively. μ is the shear modulus, γ is the stacking fault energy, and b N and b P are the magnitudes of the Burgers vectors of the perfect dislocation and the Shockley partial DS, respectively. The D is the grain size or twin thickness. From formulae (1) and (2), the critical shear stresses needed to nucleate a dislocation increases as the grain size decreases. For Ni with an stacking fault energy of 0.124–0.182 J m −2 and a shear modulus of 93.2 GPa [36] , [37] , the critical shear stresses for a full and a partial dislocation nucleation in the 6 nm thickness twin are ~11.55 GPa and 6.67–6.97 GPa, respectively. This required nucleation stress is too high to be reached in our NW. According to our ab initio calculation, the maximum shear stress along direction is ~4 GPa ( Supplementary Fig. S11 ), consistent with the results of 3.17–6.3 GPa reported in a previous work [38] . Thus, the calculated shear strength of Ni is even lower than the stresses needed for nucleating partial or full dislocations. Therefore, large lattice shear can be achieved inside the twins 1–6 nm in thickness, in the absence of nucleated dislocations. Second, due to the single crystalline nature of the wire, grain rotation can also be excluded. Third, additional twinning in these ultra-thin twin lamellae is difficult. Fourth, the bent twin platelets are confined by elastic surroundings with a large strain/stress gradient, which effectively enabled the elastic events of the FCC R lattice (with strain of 34.6%) back to BCT lattice (with strain of 17.3%) and further to the original FCC lattice. Fifth, based on our ab initio calculations, through the entire straining process, there does not exist any other energy valley for another structure (see Supplementary Fig. S11 ). An alternative strain-induced phase transition is also excluded in the lattice shearing path. With all of these and the 3D bending stress state, the bent NWs avoided all of the inelastic processes that would otherwise set in and lead to sample failure at high stresses under uniaxial tension or compression. These factors allow us, for the first time, to directly witness the entire continuous lattice deformation process to an extent far beyond the level metals can normally sustain. The phenomenon revealed in this study is different from the Bain transformation [39] , that is, the FCC to body-centred cubic (BCC) structure or BCT martensitic transformation, in which two stable or metastable phases (stress-free state) exist corresponding to two basins/valleys on the energy landscape [40] , [41] . It is also different from the observed BCC phase transitions in epitaxial thin films [42] through the Bain path, in which uni-axial tensile stress and principle-axis straining were always involved [43] , [44] , [45] . Our observation demonstrated that the lattice deformation of an FCC nanomaterial metals in tension is not always associated with the classical Bain path, but can rather be the lattice shear in the <112>{111} system [24] , [46] . In summary, using atomic-scale in situ experiments on Ni NWs inside a TEM, we have presented atomic-scale evidence that a very large lattice shear strain up to 34.6% can be sustained in a bent NW. In the confined bent nano-domains far away from dislocation disturbed regions, we observed, for the first time, the entire gradual process of continuous and reversible FCC–BCT–FCC R lattice shear evolution, which was predicted in theory but has never been experimentally verified before. The complete continuous lattice shear process can be terminated at lower shear strain values due to the intervention of dislocations. This hyper-elastic feature of Ni NWs can store an extremely high density of elastic energy—more than 100 times than that in bulk metals. These findings may lead to new nanoscale metallic materials that possess ultra-high strength and unprecedented capacity for elastic energy storage. These results also have implications for new opportunities of strain engineering to tune properties, which require large straining capability of materials. In situ bending tests details The atomic-scale in situ bending experiments of individual NWs were realised by using our recently developed method [26] , [27] . The NWs were scattered on a previously broken TEM grid, which was covered by CTFs. The scattered NWs could then be bent or deformed by tensile stress by the CTF at low strain rates (~10 −4 s −1 ) (See Supplementary Movie 1 ). With this method, the specimen could tilt along two orthogonal directions by large angles (±20°) with no special specimen holder or mechanical tensile attachments. Thus, along an optional direction, the bending or axial tensile deformation of individual NWs can be in situ recorded at the atomic scale. The experiments were carried out using a JEOL HRTEM with a field-emission gun (JEOL 2010 F). The point resolution was 0.19 nm. The geometrical phase analysis The GPA is a powerful method to generate quantitative shear strain maps from standard HRTEM images [28] . For an HRTEM lattice image, the two-dimensional (2D) lattice is characterized by the presence of strong Bragg reflections in its Fourier transform pattern. The GPA technique is based on combining real-space and Fourier-space information. Choosing two reciprocal lattice vectors (Bragg reflections) in the Fourier transform of a reference region implicitly defines a 2D lattice in the HREM image, and then the strain can be measured by calculating the Fourier components of the lattice in an image [28] . With this technique, the local structure variation in terms of strains can be mapped from the HRTEM image. In this study, the shear strain was defined by . During strain field calculation, the reference region of zero-strain was defined in the inner part of the red boxes (see Fig. 3a ), and the colours in the map show the relative shear strain compared with the red framed region of Fig. 3a . The quantitative strain profile was extracted from the coloured strain maps using intensity line scanning with the line width of 0.5 nm. Simulation details Ab initio simulations were conducted using the Vienna ab initi o simulation package (VASP) [47] . The projected augmented wave method [48] and the generalized gradient approximation were used to describe the electron–ion interaction [49] . A thermal broadening of 0.02 eV was applied to improve the convergence of the self-consistent procedure, and non-spin polarization was employed in all calculations. For bulk FCC Ni, a 20 × 20 × 20 Monkhorst–Pack grid was used to integrate over the Brillouin zone of the elemental FCC unit cell, and the equilibrium lattice constant for FCC Ni was calculated to be 3.49 Å, which is in good agreement with that determined by experiment (3.524 Å). To investigate the deformation of FCC Ni along the direction, a supercell was employed (as shown in Fig. 4a ), and a dense k-point grid (30 × 30 × 30) was used for the structure relaxation and total energy calculation. In order to simulate the uniaxial tensile and shear, we applied quasi-continuous strains to the simulated systems and fully relaxed the stressed cells with pre-set applied strain. For the shear deformation, we applied pure shear to the simulated systems and the engineering shear strain was defined by: . The components of stress tensors corresponding to the loading direction were set to zero during relaxation. For example, the is set to zero for uniaxial tension in the ( x ) direction and for shear along ( xy ) plane. The total energy was calculated based on the finally relaxed atomic configuration at each applied strain, ɛ . How to cite this article: Wang, L. et al. In situ atomic-scale observation of continuous and reversible lattice deformation beyond the elastic limit. Nat. Commun. 4:2413 doi: 10.1038/ncomms3413 (2013).